Disparity between microRNA levels and promoter strength is associated with initiation rate and Pol II pausing MicroRNAs are transcribed by RNA polymerase II but the transcriptional features influencing their synthesis are poorly defined. Here we report that a TATA box in microRNA and protein-coding genes is associated with increased sensitivity to slow RNA polymerase II. Promoters driven by TATA box or NF-κB elicit high re-initiation rates, but paradoxically lower microRNA levels. MicroRNA synthesis becomes more productive by decreasing the initiation rate, but less productive when the re-initiation rate increases. This phenomenon is associated with a delay in miR-146a induction by NF-κB. Finally, we demonstrate that microRNAs are remarkably strong pause sites. Our findings suggest that lower efficiency of microRNA synthesis directed by TATA box or NF-κB is a consequence of frequent transcription initiations that lead to RNA polymerase II crowding at pause sites, thereby increasing the chance of collision and premature termination. These findings highlight the importance of the transcription initiation mechanism for microRNA synthesis, and have implications for TATA-box promoters in general. MicroRNAs (miRNAs) are a class of noncoding RNAs that regulate stability and translation of target mRNAs [1] . miRNAs are important regulators in many physiological processes and their misexpression has been found to be associated with a variety of diseases [2] . A miRNA is synthesized as a long primary transcript (pri-miRNA) that is cleaved in the nucleus by the RNase Drosha to produce pre-miRNA, an ~70-nucleotide molecule containing a characteristic stem-loop structure. The pre-miRNA is transported to the cytoplasm, and is further processed by the RNase Dicer into mature miRNA. miRNAs are either encoded by autonomous genes, or are processed from various RNA sources such as introns, 3′ UTRs and long noncoding RNAs [1] . Most miRNAs are transcribed by RNA polymerase II (PolII) [3] , [4] and recent studies suggest that nuclear processing of the pri-miRNA by Drosha is coupled to transcription [5] . However, the potential effect of the transcription initiation process, through different promoters, on miRNA synthesis is presently unknown. Regulation of transcription of protein-coding and noncoding genes is governed by two types of cis-regulatory elements known as enhancers and core promoters. The core promoter consists of sequence elements that surround the transcription start site (TSS), and serve as a docking site for general transcription factors and PolII that assemble into a pre-initiation complex (PIC) [6] , [7] . The core promoter has a crucial role in transcription, as it functions as the most important target for enhancer-bound transcription factors; it contributes to the overall efficiency of the transcription process and determines the site of transcription initiation. The TATA box, which is the first core promoter element to be identified and characterized in eukaryotes [8] , has a strict location between (−35) and (−25) relative to the TSS. It is present in a fraction of PolII genes: between 20 and 46% in yeast (depending on the definition of the TATA-box sequence) [9] , [10] , ~30% of Drosophila genes [11] and up to ~20% of human genes [12] , [13] , [14] , [15] . The presence or absence of a TATA box in core promoters has been linked in yeast [9] , [10] , [16] , [17] , [18] and humans [19] to two pathways of PIC assembly, one being TFIID-dependent (weak TATA or TATA-less) and the other TFIID-independent and SAGA dependent, suggesting that the mechanism of transcription initiation in TATA-less promoters is quite different from TATA promoters [20] . Bioinformatics analysis of human genes has revealed a surprising observation: genes with a TATA box are much shorter than TATA-less genes. Furthermore, within the TATA-containing genes, length is inversely correlated to the strength of the TATA box [14] . Analysis of gene expression data revealed the expected inverse correlation between gene length and levels of expression, but this negative correlation is the highest for genes with a TATA box and lowest for TATA-less genes. Having a TATA box in the core promoter seems beneficial for expression of short genes, while its advantage diminishes with longer genes. The underlying basis for this phenomenon is presently unknown. In the present study, we examined the influence of specific promoter features and of elongation dynamics on the efficiency of miRNA synthesis. Our findings stress the importance of the transcription initiation mechanism in determining the efficiency of co-transcriptional miRNA processing. Genes affected by slow PolII are enriched with a TATA box To investigate the influence of elongation rate on gene expression, we used the α-amanitin-resistant human PolII large subunit (Rpb1-am r ) and a mutated variant (R749H-am r ) that exhibits a slower elongation rate in vitro and in vivo [21] , [22] , [23] . Cells were transfected with plasmids encoding the α-amanitin-resistant variants of PolII and 24 h later selected for the expression and function of the exogenous Rpb1 by incubation with α-amanitin. After additional 24 h, global gene expression changes were determined using microarray chips. Within the time frame of the experiment (24 h), 167 genes were reproducibly downregulated in the R749H-am r compared with Rpb1-am r -expressing cells, in three independent experiments ( Supplementary Data 1 ). We selected six genes for validation using quantitative real-time RT–PCR analysis and found that all the selected genes were indeed downregulated and to a greater extent than the microarray ( Fig. 1a ). Analysis of the genomic structure of the affected genes revealed significant enrichment of long genes with their median length ~1.6-fold higher than that of all expressed genes ( Fig. 1b , left). The enrichment of long genes is accompanied with an increase in the number of exons ( Fig. 1b , middle). We also analysed the expression levels and found that the affected genes are typically expressed at higher levels compared with all expressed genes in the microarray ( Fig. 1b , right). The enrichment of long genes is expected due to accumulation of transcriptional elongation delay, confirming that the R749H-am r is slow. However, ~37% of the downregulated genes are nevertheless relatively short (>27,405 bp, the median length of all expressed genes) ( Fig. 1c ), with a particular enrichment of the intron-less histone genes, which are among the shortest genes in mammalian cells ( Supplementary Data 1 ). To examine whether the sensitivity of the short genes to the slow PolII is associated with other transcription regulatory features, we analysed their promoters. Remarkably, the majority of the short genes (67%) are governed by TATA-box promoter (TATAA with up to one mismatch at the appropriate location) ( Fig. 1c ), which is eightfold higher than the prevalence of the TATA box is all genes (8.3%,) and fivefold higher than the prevalence in short genes (12.5%) [14] . The enrichment of the TATA box persists even without the histone genes (45%) and is also seen among the affected long genes. These findings raise the possibility that a TATA promoter may confer susceptibility to a slow rate of elongation. 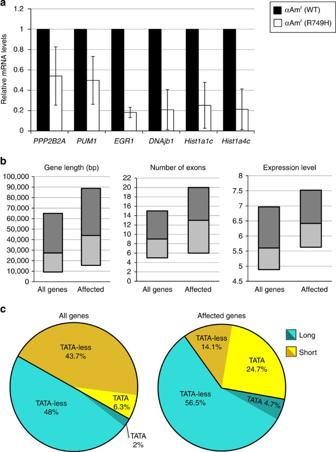Figure 1: Enrichment of TATA-box promoter among short genes affected by a slow RNA polymerase II. HEK293T cells were transfected with the Rpb1-amror slow (R729H-amr) α-amanitin-resistant subunit of RNA PolII and selected with α-amanitin 24 h after transfection for an additional 24 h. Total RNA was extracted and global changes in gene expression were determined using microarray chips. (a) From the list of affected genes (Supplementary Data 1), six genes were selected for validation using RT–qPCR. The results were normalized to the mRNA levels of GAPDH. The level of the transcript in cells expressing the WT α-amanitin-resistant PolII was set to 1. The graph represents the mean of three independent transfection experiments. Error bars represent standard error (s.e.). (b) Gene length, exons number and expression level of the affected genes. Gene length and exon number of all expressed genes and the genes affected by the slow RNA PolII were retrieved from the UCSC genome browser. Expression levels are derived from the microarray results. The data are presented as boxplots that show the 25%, median and 75% quartile values for each gene set. (c) Pie charts that show the distribution of all genes or genes affected by the slow RNA PolII according to their length (greater or smaller than the median length in all genes). Long genes are in blue and short in yellow. Each group is further divided into TATA and TATA-less genes. The promoter sequence for each gene was retrieved from the DBTSS, and a gene was considered TATA if the TATA-box (TATAA with up to 1 mismatch) is present 20–35 nucleotides upstream of the TSS. Figure 1: Enrichment of TATA-box promoter among short genes affected by a slow RNA polymerase II. HEK293T cells were transfected with the Rpb1-am r or slow (R729H-am r ) α-amanitin-resistant subunit of RNA PolII and selected with α-amanitin 24 h after transfection for an additional 24 h. Total RNA was extracted and global changes in gene expression were determined using microarray chips. ( a ) From the list of affected genes ( Supplementary Data 1 ), six genes were selected for validation using RT–qPCR. The results were normalized to the mRNA levels of GAPDH. The level of the transcript in cells expressing the WT α-amanitin-resistant PolII was set to 1. The graph represents the mean of three independent transfection experiments. Error bars represent standard error (s.e.). ( b ) Gene length, exons number and expression level of the affected genes. Gene length and exon number of all expressed genes and the genes affected by the slow RNA PolII were retrieved from the UCSC genome browser. Expression levels are derived from the microarray results. The data are presented as boxplots that show the 25%, median and 75% quartile values for each gene set. ( c ) Pie charts that show the distribution of all genes or genes affected by the slow RNA PolII according to their length (greater or smaller than the median length in all genes). Long genes are in blue and short in yellow. Each group is further divided into TATA and TATA-less genes. The promoter sequence for each gene was retrieved from the DBTSS, and a gene was considered TATA if the TATA-box (TATAA with up to 1 mismatch) is present 20–35 nucleotides upstream of the TSS. Full size image TATA-box miRNA genes are more susceptible to slow PolII We next examined the effect of elongation rate on expression of miRNAs and its relation with transcription regulatory features. We selected a subset of miRNAs on the basis of experimentally mapped TSS position, which allows the definition of the promoter; expression of the miRNA in the cells; and qualification of the miRNA for RT–qPCR analysis. Supplementary Table S1 shows a list of miRNA genes with validated TSSs that we collected either from the literature or from public databases. It is evident from this data that miRNA genes with TATA promoters constitute a very small group, consistent with the low prevalence of the TATA box in general [14] . We analysed the effect of the α-amanitin-resistant slow PolII mutant R749H-am r described above on levels of native miRNAs, measured by quantitative real-time PCR and normalized to the PolIII-dependent U6 RNA ( Fig. 2 ). In analysing the data, we also took into consideration the distance between the TSS and the miRNA-coding sequence, as the susceptibility to a slow PolII is expected to be proportional to the length of the transcript. As expected, miRNAs located tens of kilobases away from the TSS, miR-107 , miR-30e , miR-32 and miR-339 , were downregulated by the slow Rpb1, most likely due to increased transcription elongation delay. With miRNAs localized closer to the TSS, the slow PolII significantly diminished the expression of miR-554 and miR-590 , while it hardly affected the expression of miR-15b , and miR-23a , miR-423 , miR-616 , miR-22, miR-15b, miR-148b, miR-643 and miR-631 ( Fig. 2 ). Interestingly, the two miRNAs that were affected by the slow PolII are the only ones driven by TATA-box promoters, whereas the unaffected miRNAs were all TATA-less. Thus, the sensitivity to a slow rate of elongation in short miRNA genes, seems to correlate with a TATA box as was observed with the protein-coding genes. 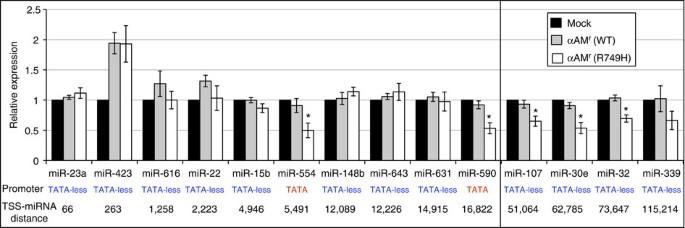Figure 2: A slow RNA polymerase II differentially affect expression of endogenous miRNAs. HEK293T cells were transfected with the Rpb1-amror slow (R729H-amr) α-amanitin-resistant subunit of RNA PolII and selected with α-amanitin. Total RNA was extracted and the levels of endogenous miRNAs were determined using RT–qPCR specific for miRNA (seeMethods). The miRNAs were selected according to the criteria described in the results section fromSupplementary Table S1. Core promoter type and the distance from the TSS of each miRNA are indicated. miRNA levels in mock transfected cells was set to 1. The graph represents the mean of three independent transfection experiments and error bars represent s.e. The asterisk indicates a statistically significant difference (P<0.05, Student’st-test). Figure 2: A slow RNA polymerase II differentially affect expression of endogenous miRNAs. HEK293T cells were transfected with the Rpb1-am r or slow (R729H-am r ) α-amanitin-resistant subunit of RNA PolII and selected with α-amanitin. Total RNA was extracted and the levels of endogenous miRNAs were determined using RT–qPCR specific for miRNA (see Methods ). The miRNAs were selected according to the criteria described in the results section from Supplementary Table S1 . Core promoter type and the distance from the TSS of each miRNA are indicated. miRNA levels in mock transfected cells was set to 1. The graph represents the mean of three independent transfection experiments and error bars represent s.e. The asterisk indicates a statistically significant difference ( P <0.05, Student’s t -test). Full size image Disparity between TATA-box promoter activity and miRNA level To investigate further the potential link between promoter features and miRNA expression, we selected the mir-22 gene for further analysis, as it is comprised of a strong ubiquitous TATA-less promoter confined to ~500 nt upstream of the TSS [24] . The gene has three exons and the pre-miR-22 is processed from the second exon. We constructed a miR-22 mini-gene (MG) in which the promoter, the first two exons and part of the intron were placed upstream of the luciferase gene ( Fig. 3d ). Another MG variant (MG-Δpre) is similar to the MG except that the pre-miR-22 and flanking sequences were deleted from the second exon ( Fig. 3b ), as they dramatically reduced the luciferase expression from the MG due to miRNA processing ( Fig. 3f ). In addition, we used a construct containing only the miR-22 promoter ( Fig. 3a ). We next introduced a canonical TATA box (TATAAAA) to the miR-22 promoter by altering the nucleotide sequence at positions −35 to −28, relative to the TSS by direct mutagenesis. The mutation was introduced into the three types of reporter genes: the promoter-luciferase reporter, the MG without the pre-miRNA (Δpre) and the intact MG. As expected, the addition of a TATA box enhanced the luciferase activity directed by the miR-22 promoter by approximately threefold, both in the promoter-luciferase and in the Δpre-MG context ( Fig. 3a ). A similar enhancement in promoter activity was also measured at the mRNA level transcribed from the Δpre-MG using a northern blot of luciferase mRNA ( Fig. 3c ), confirming that the luciferase assay is a faithful measure of promoter activity, and that the TATA-box effect on transcription is independent of splicing. To assess the efficiency of miRNA synthesis directed by the TATA-less and TATA versions of the miR-22 promoter, cells were transfected with the intact miR-22 MGs and 48 h later miRNA levels were determined by northern blot analysis of small RNAs. We normalized for transfection efficiency and sample preparation by co-transfecting into the cells an expression plasmid directing the synthesis of a 42-nucleotide-long small RNA of a randomly chosen sequence, under the control of the H1 PolIII promoter. As shown in Fig. 3d , the three- to fourfold enhancement in promoter strength conferred by the TATA box is reduced to only a 1.4-fold enhancement of miRNA expression, suggesting that the efficiency of miRNA synthesis is reduced when transcription initiation is directed by a TATA box. We examined the effect of miR-22 expressed from the MGs on its known target PTEN [24] , [25] , [26] , [27] , [28] and found the reduction in PTEN reflects the level of expression of the miRNA ( Supplementary Fig. S1 ). One possibility to explain this phenomenon may be inefficient recruitment of miRNA-processing factors to the TATA-driven gene. According to this possibility, the cleavage of the primary transcript by Drosha would be less efficient and consequently expression of the downstream luciferase should increase. However, we found that the luciferase expression (read-through) directed by the TATA promoter from the intact MGs is inhibited to an even greater extent compared with the TATA-less counterpart ( Fig. 3f , compare left and middle columns), rendering this possibility unlikely. In fact the read-through luciferase activity reflect the level of the miRNA. 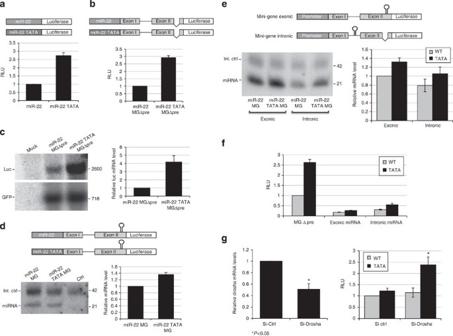Figure 3: miRNA expression directed by a TATA box is not correlated with promoter strength. (a) The miR-22 promoter and its TATA-box derivative were transfected into HEK293T together with RSV-Renillaand 24 h later luciferase activities were determined. The results represent the mean of 15 independent experiments and error bars represent s.e. (b) A MG derived from themiR-22gene as schematically shown, was cloned upstream to a luciferase reporter gene. To allow luciferase production, the pre-miRNA sequence was removed (Δpre). The luciferase activity of the WT and TATA MGs was determined from eight independent transfection experiments. (c) The WT and TATA Δpre miR-22 MG constructs were co-transfected with CMV-GFP into HEK293T and 48 h later the levels of luciferase and GFP mRNAs were measured by northern blot. A representative autoradiogram and a graph representing the mean of two independent repeats are shown. Error bars represent standard deviation (s.d.). (d) The WT and TATA intact miR-22 MGs were co-transfected into HEK293T together with a control plasmid expressing a small noncoding RNA under the H1 promoter. At 48 h, the miR-22 and the internal control levels were measured by northern blot of small RNAs. A representative autoradiogram and a graph representing the mean of nine independent repeats are shown. Error bars represent s.e. (e) Exonic or intronic miRNAs constructs were transfected into HEK293T and miR-22 and control RNA levels were determined by northern blot 48 h later. Representative autoradiogram and graph presenting the mean of five independent repeats are shown. Error bars represent s.e. (f) The intact exonic and intronic and the Δpre MG constructs (WT or TATA) were transfected into cells and luciferase levels were measured. The graph represents mean of six independent repeats. Error bars represent s.e. (g) HEK293T cells were transfected with control or Drosha-specific siRNA and 48 h later cells were transfected again with the WT and TATA intact MG constructs together RSV-Renilla. After 24 h, Drosha and GAPDH mRNA levels were analysed by RT–qPCR (left panel) in parallel to firefly andRenillaluciferase activities (right panel). In all sections, the level directed by the WT miR-22 promoter was set to 1. The graph represents mean of three independent repeats. Error bars represent s.e. The asterisk indicates a statistically significant difference (P<0.05, Student'st-test). Figure 3: miRNA expression directed by a TATA box is not correlated with promoter strength. ( a ) The miR-22 promoter and its TATA-box derivative were transfected into HEK293T together with RSV- Renilla and 24 h later luciferase activities were determined. The results represent the mean of 15 independent experiments and error bars represent s.e. ( b ) A MG derived from the miR-22 gene as schematically shown, was cloned upstream to a luciferase reporter gene. To allow luciferase production, the pre-miRNA sequence was removed (Δpre). The luciferase activity of the WT and TATA MGs was determined from eight independent transfection experiments. ( c ) The WT and TATA Δpre miR-22 MG constructs were co-transfected with CMV-GFP into HEK293T and 48 h later the levels of luciferase and GFP mRNAs were measured by northern blot. A representative autoradiogram and a graph representing the mean of two independent repeats are shown. Error bars represent standard deviation (s.d.). ( d ) The WT and TATA intact miR-22 MGs were co-transfected into HEK293T together with a control plasmid expressing a small noncoding RNA under the H1 promoter. At 48 h, the miR-22 and the internal control levels were measured by northern blot of small RNAs. A representative autoradiogram and a graph representing the mean of nine independent repeats are shown. Error bars represent s.e. ( e ) Exonic or intronic miRNAs constructs were transfected into HEK293T and miR-22 and control RNA levels were determined by northern blot 48 h later. Representative autoradiogram and graph presenting the mean of five independent repeats are shown. Error bars represent s.e. ( f ) The intact exonic and intronic and the Δpre MG constructs (WT or TATA) were transfected into cells and luciferase levels were measured. The graph represents mean of six independent repeats. Error bars represent s.e. ( g ) HEK293T cells were transfected with control or Drosha-specific siRNA and 48 h later cells were transfected again with the WT and TATA intact MG constructs together RSV- Renilla . After 24 h, Drosha and GAPDH mRNA levels were analysed by RT–qPCR (left panel) in parallel to firefly and Renilla luciferase activities (right panel). In all sections, the level directed by the WT miR-22 promoter was set to 1. The graph represents mean of three independent repeats. Error bars represent s.e. The asterisk indicates a statistically significant difference ( P <0.05, Student's t -test). Full size image Many miRNA genes are embedded within introns, whereas the miR-22 gene is exonic. The differential effect of TATA-less and TATA promoter on miRNA synthesis may be linked to the location from which it is processed. To address the influence of the miRNA location, and whether it is associated with the differential effect of core promoter type, we constructed another set of MGs in which the pre-miR-22 and its flanking sequences were removed from the exon and placed in the middle of the intron. The exonic and intronic miRNA-expressing plasmids were transfected into cells and the miRNA levels monitored by northern blot. Expression from the intronic site is less efficient than from the exonic site ( Fig. 3e ), however the relative activities of the TATA and TATA-less promoters on miRNA expression was similar in both locations, indicating that reduced efficiency of miRNA processing associated with the TATA-box is not linked to its location. Analysis of the luciferase activity (read-through) expressed from the intronic constructs revealed reduction in luciferase levels compared with the Δpre constructs, but higher levels relative to the exonic constructs ( Fig. 3f ), suggesting that in this specific arrangement of the MG splicing and miRNA synthesis are competitive. To determine whether the reduction in productive expression of the miRNA as well as the read-through luciferase, are a consequence of the nuclear processing of the miRNA, cells were transfected with siRNA against Drosha, the initiating miRNA-processing enzyme. At 48 h after transfection, the cells were transfected again with the intact MGs described above. Analysis of Drosha mRNA levels by RT–qPCR confirms its partial depletion by the specific but not the control siRNA ( Fig. 3g , left panel). As Drosha is expected to affect miRNA synthesis, we examined the levels of the read-through luciferase, which reflect the efficiency of miRNA synthesis. Downregulation of Drosha partially restored the correlation between promoter strength and the read-through luciferase levels ( Fig. 3g , right panel), suggesting that the processing of the miRNA by Drosha is involved in this phenomenon. The TATA box is more susceptible to slow PolII Considering that the effect of a slow elongating PolII on endogenous miRNAs and mRNA genes is correlated with the presence of a TATA box ( Figs 1 and 2 ), we next wished to examine more directly the interplay between core promoter type and elongation dynamics. For this purpose, cells were transfected with the plasmids encoding the α-amanitin-resistant variants of PolII together with the miR-22 MGs under the control of the wild-type miR-22 promoter or the TATA-box version. Following α-amanitin selection, the miRNA levels were analysed by northern blot. As the internal control RNA is transcribed by PolIII, it is not expected to be affected by the α-amanitin dose used here. The results revealed that following α-amanitin treatment, there was a similar ~80% recovery of miRNA expression by the α-amanitin-resistant PolII from the two promoters, as compared with untreated cells ( Fig. 4a , compare lanes 7 and 9 with 4 and 5). The slow elongating PolII, on the other hand, had differential effect; it restored ~40% of the miRNA expression directed by the WT miR-22 ( Fig. 4a , compare lanes 5 and 10 and Fig. 4b ), but only 13% of miRNA directed by the TATA-box promoter ( Fig. 4a , compare lanes 4 and 8 and Fig. 4b ). In fact with the slow elongating PolII, the activity of the native miR-22 promoter is even twofold higher than that of the TATA promoter, which is the opposite from the relative activity with the WT PolII or untreated cells ( Fig. 4b ). These results suggest that transcription directed by the TATA box is indeed more sensitive to interruptions during elongation, which is in line with the effect of the slow PolII on endogenous miRNAs driven by a TATA box. 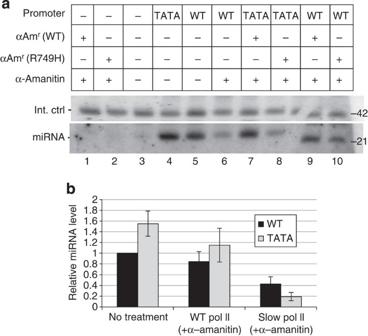Figure 4: A slow polymerase differentially affects TATA and TATA-less promoters. (a) The MG constructs under the regulation of miR-22 WT or TATA promoters were co-transfected with the internal control plasmid, and either Rpb1-amror slow (R729H-amr) α-amanitin-resistant subunit of RNA PolII, into HEK293T. After 24 h, cell medium was replaced with fresh (lanes 3–5) or α-amanitin-containing medium (lanes 1–2 and 6–10). At 48 h post transfection, RNA was extracted, and miR-22 and internal control levels were measured by northern blot. A representative autoradiogram of the northern blot is shown. (b) The graph represents the mean of four independent experiments as shown ina. Error bars represent s.e. The miRNA level directed by the WT miR-22 promoter in untreated cells was set to 1. Figure 4: A slow polymerase differentially affects TATA and TATA-less promoters. ( a ) The MG constructs under the regulation of miR-22 WT or TATA promoters were co-transfected with the internal control plasmid, and either Rpb1-am r or slow (R729H-am r ) α-amanitin-resistant subunit of RNA PolII, into HEK293T. After 24 h, cell medium was replaced with fresh (lanes 3–5) or α-amanitin-containing medium (lanes 1–2 and 6–10). At 48 h post transfection, RNA was extracted, and miR-22 and internal control levels were measured by northern blot. A representative autoradiogram of the northern blot is shown. ( b ) The graph represents the mean of four independent experiments as shown in a . Error bars represent s.e. The miRNA level directed by the WT miR-22 promoter in untreated cells was set to 1. Full size image We also measured the influence of the slow PolII on the read-through luciferase activity and found that the α-amanitin-resistant PolII failed to effectively restore the luciferase activity in both constructs ( Supplementary Fig. S2A ), which differ from the effect on the miRNA expression ( Fig. 4 ). We therefore examined whether the miRNA synthesis is involved by analysing the constructs lacking the miRNA (Δpre). The same effect was apparent with the Δpre constructs, as the α-amanitin-resistant PolII variants did not efficiently rescued the luciferase expression ( Supplementary Fig. S2B ). These findings suggest that the α-amanitin-resistant mutants have also post-transcriptional effects. Notably, the expression of the exogenous miR-22 appears to be more dramatically affected by the α-amanitin-resistant PolII variants than the endogenous miR-22 ( Fig. 2 ). This difference likely reflects the fact that only a portion of the endogenous miR-22 that we measured is actually transcribed by the transfected polymerases during course of the α-amanitin treatment (24 h), as the half lives of miRNAs is very long [29] , [30] , [31] . In contrast, most of the exogenous miR-22 is being newly synthesized during the experiment. Productive miRNA synthesis is restored by lower initiation rate Transcription directed by TATA-box promoters, but not through TATA-less promoters, is produced through re-initiation [32] or bursts [33] . This raises the possibility that a high frequency of transcription initiation is incompatible with efficient miRNA expression. To test this prediction, we first examined whether the introduction of a TATA box in the miR-22 promoter enhanced the rate of re-initiation by using in vitro transcription assays. The WT and the TATA version of the miR-22 promoter were each incubated with nuclear extract together with a GFP reporter plasmid that served as internal control. After 30 min incubation that allowed the formation of the PIC, transcription was initiated by the addition of NTPs and the reaction proceeded for 10 min. Subsequently, the correctly initiated transcript was analysed by a modified 5′RACE (see Methods ). To examine the occurrence of transcription re-initiation, we used the detergent Sarkosyl, which is known to inhibit initiation but not elongation [34] . If Sarkosyl is added soon after initiation, it allows completion of the already initiated transcripts but prevents subsequent transcription initiation cycles. 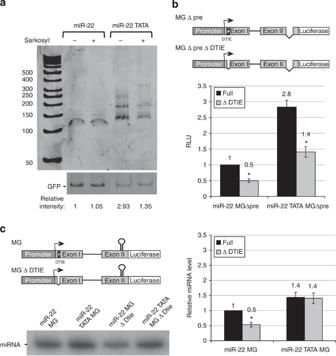Figure 5: Reduction of transcription initiation rate restores the correlation between promoter activity and miRNA synthesis. (a) The TATA box increases re-initiation rate.Luciferasereporter gene under the WT and TATA versions of the miR-22 promoter, were incubated with nuclear extract for 30 min to let the PIC form. CMV-GFP plasmid, which served as internal control, was also included in the reaction. Transcription was initiated by addition of NTPs. Sarkosyl was added shortly after initiation to eliminate re-initiation. Transcripts were analysed by 5′RACE as described in the Methods section. The PCR products were run on 6% PAGE and stained with ethidium bromide. The relative intensity of the products was determined by densitometry and shown in the bottom. (b) DTIE was deleted from either the WT or TATA versions of the miR-22 promoter in the Δpre MG context and transfected into HEK293T together with RSV-Renilla. After 24 h, the relative luciferase activities were determined. The results represent the mean of three independent transfection experiments and the error bars represent s.e. (c) DTIE was deleted from the WT or TATA versions of the miR-22 promoter in the context of the intact MG and then co-transfected into HEK293T cells with a plasmid directing the expression of secretedRenilla luciferaseto control for transfection efficiency. At 48 h post transfection, the medium was collected forRenilla luciferaseactivity measurements, RNA was extracted from the cells and the level of the miRNA was measured by northern blot. A representative autoradiogram of the northern blot is shown. The graph represents the mean of three independent experiments and error bars represent s.e. In all sections, the level directed by the WT miR-22 promoter was set to 1. The asterisks indicate a statistically significant difference (P<0.05, Student'st-test). Figure 5a shows the correctly initiated transcripts directed by the WT and the TATA versions of the miR-22 promoters. The 5′RACE products directed by the WT and the TATA promoters differ slightly in their size, as the TSS directed by the TATA is located 7 nucleotides upstream relative to the WT TSS. The activity of the miR-22-TATA promoter is clearly sensitive to inhibition by Sarkosyl, while the WT TATA-less promoter is not ( Fig. 5a ), confirming that during the course of the experiment the TATA-box promoter directed several rounds of initiations. Figure 5: Reduction of transcription initiation rate restores the correlation between promoter activity and miRNA synthesis. ( a ) The TATA box increases re-initiation rate. Luciferase reporter gene under the WT and TATA versions of the miR-22 promoter, were incubated with nuclear extract for 30 min to let the PIC form. CMV-GFP plasmid, which served as internal control, was also included in the reaction. Transcription was initiated by addition of NTPs. Sarkosyl was added shortly after initiation to eliminate re-initiation. Transcripts were analysed by 5′RACE as described in the Methods section. The PCR products were run on 6% PAGE and stained with ethidium bromide. The relative intensity of the products was determined by densitometry and shown in the bottom. ( b ) DTIE was deleted from either the WT or TATA versions of the miR-22 promoter in the Δpre MG context and transfected into HEK293T together with RSV- Renilla . After 24 h, the relative luciferase activities were determined. The results represent the mean of three independent transfection experiments and the error bars represent s.e. ( c ) DTIE was deleted from the WT or TATA versions of the miR-22 promoter in the context of the intact MG and then co-transfected into HEK293T cells with a plasmid directing the expression of secreted Renilla luciferase to control for transfection efficiency. At 48 h post transfection, the medium was collected for Renilla luciferase activity measurements, RNA was extracted from the cells and the level of the miRNA was measured by northern blot. A representative autoradiogram of the northern blot is shown. The graph represents the mean of three independent experiments and error bars represent s.e. In all sections, the level directed by the WT miR-22 promoter was set to 1. The asterisks indicate a statistically significant difference ( P <0.05, Student's t -test). Full size image Next, we set out to examine how modulation of transcription initiation affects productive miRNA synthesis. We have identified a regulatory element within the miR-22 promoter located between +23 and +31 relative to the TSS that we named downstream transcription initiation element (DTIE). This element consists of a novel sequence and influences both transcription level and TSS location, reminiscent of a transcription initiation element (Marbach-Bar et al ., manuscript in preparation). We therefore used DTIE to modulate the transcription initiation rate of the MGs. We created DTIE deletions both in the WT and TATA miR-22 promoters either in the Δpre or in the intact MG contexts ( Fig. 5b and c ). Deletion of DTIE reduced the luciferase activity of the Δpre MGs directed by both the WT and the TATA promoters by ~50% ( Fig. 5b ). Note that the strength of the TATA promoter without DTIE is 1.4-fold higher than the native promoter. Next, we determined the level of miRNA synthesis and found that the amount directed by the native miR-22 promoter was reduced by 50% upon DTIE deletion ( Fig. 5c ), similar to the effect on the luciferase levels. As before, the relative amount of the miRNA driven by the TATA-box promoter is only 1.4, which is a reduction compared with the 2.8 measured in the luciferase assay. Interestingly, the miRNA level driven by the miR-22-TATA without DTIE is also 1.4, and this level exactly matches the relative promoter strength measured in Fig. 5b . Thus, reducing the initiation rate in the TATA promoter through deletion of DTIE restored the correlation between promoter strength and miRNA expression, which is an indication that miRNA synthesis becomes productive. miRNA synthesis is sensitive to high rate of re-initiation If high transcription initiation rate reduces the efficiency of miRNA expression, we expect that raising the initiation rate would diminish the efficiency of miRNA production regardless of core promoter type. To gain evidence for this notion, we utilized the TATA-less A20 promoter, which is a direct target for the inducible transcription factor NF-κB. We have previously shown that one of the effects of NF-κB on A20 gene transcription is stimulation of re-initiation [35] . To validate these findings, we performed in vitro transcription assays with nuclear extracts prepared from control cells or cells treated with the cytokine TNFα, a potent NF-κB inducer. As shown in Supplementary Fig. S2 , the basal activity of A20 promoter is resistant to inhibition by Sarkosyl, whereas the TNFα-induced transcription is sensitive to Sarkosyl, confirming that activation of the A20 promoter by NF-κB involves enhancement of re-initiation. To examine the effect of NF-κB on miRNA expression, the A20 promoter was inserted upstream to the Δpre or the intact MGs described above. Cells were transfected with either the Δpre or the intact MG under the control of the A20 and miR-22 promoters and then NF-κB activity was induced by TNFα. The miR-22 promoter is stronger than the A20 promoter, and upon NF-κB activation by TNFα, the luciferase activity driven by the A20 promoter was enhanced by approximately twofold, while that of miR-22 was almost unchanged ( Fig. 6a ). Under basal conditions, the level of the miRNA expression directed by the A20 promoter relative to the miR-22 promoter is maintained, however the NF-κB-induced activity of A20 is totally lost upon transcribing the miRNA ( Fig. 6b ), suggesting that miRNA synthesis is particularly sensitive to transcription occurring through re-initiation. 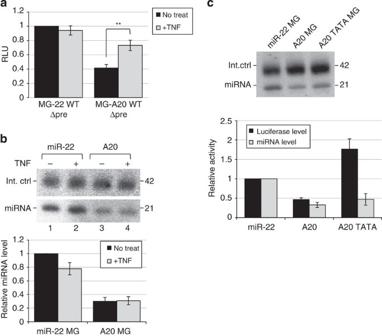Figure 6: The effect of NF-κB-induced transcription re-initiation on the efficiency of miRNA synthesis. (a) Plasmids encoding Δpre luciferase reporter MG under the control of miR-22 and A20 promoters were transfected into HEK293T together with the RSV-Renillaluciferase. At 24 h after transfection cells were induced with TNFα (20 ng ml−1) for 4 h, then cells were harvested and luciferase activity was determined. The results represent the mean of three independent transfection experiments. Error bars represent s.e. (b) Plasmids encoding the intact MG driven by the miR-22 and A20 promoters were transfected into HEK293T cells together with the internal control plasmid. At 48 h after transfection, cells were treated with TNFα for 3 h followed by RNA extraction and northern blot analysis. A representative autoradiogram of the northern blot is shown. The graph represents the mean of three independent experiments. Error bars represent s.e. (c) Comparison between the activities of the miR-22 promoter to the A20 promoter, and a mutated version of the A20 promoter (A20-TATA) that was converted into a TATA-box promoter by two point mutations19. The relative luciferase activities, driven by the different promoters in the MG context, are shown on the bottom panel as a mean of eight independent repeats and are represented by the black bars. An intact MG under the control of the indicated promoters was used to compare miRNA production directed by the different promoters. The MGs were co-transfected into HEK293T together with the control plasmid and 48 h later miRNA levels were measured by northern blot. The upper panel shows a representative northern blot autoradiogram and the graph on the bottom (grey bars) represents the mean of five independent transfection experiments. Error bars represent s.e. In all sections, the level directed by the WT miR-22 promoter was set to 1. The double asterisk indicates a statistically significant difference (P<0.001, Student'st-test). Figure 6: The effect of NF-κB-induced transcription re-initiation on the efficiency of miRNA synthesis. ( a ) Plasmids encoding Δpre luciferase reporter MG under the control of miR-22 and A20 promoters were transfected into HEK293T together with the RSV- Renilla luciferase. At 24 h after transfection cells were induced with TNFα (20 ng ml −1 ) for 4 h, then cells were harvested and luciferase activity was determined. The results represent the mean of three independent transfection experiments. Error bars represent s.e. ( b ) Plasmids encoding the intact MG driven by the miR-22 and A20 promoters were transfected into HEK293T cells together with the internal control plasmid. At 48 h after transfection, cells were treated with TNFα for 3 h followed by RNA extraction and northern blot analysis. A representative autoradiogram of the northern blot is shown. The graph represents the mean of three independent experiments. Error bars represent s.e. ( c ) Comparison between the activities of the miR-22 promoter to the A20 promoter, and a mutated version of the A20 promoter (A20-TATA) that was converted into a TATA-box promoter by two point mutations [19] . The relative luciferase activities, driven by the different promoters in the MG context, are shown on the bottom panel as a mean of eight independent repeats and are represented by the black bars. An intact MG under the control of the indicated promoters was used to compare miRNA production directed by the different promoters. The MGs were co-transfected into HEK293T together with the control plasmid and 48 h later miRNA levels were measured by northern blot. The upper panel shows a representative northern blot autoradiogram and the graph on the bottom (grey bars) represents the mean of five independent transfection experiments. Error bars represent s.e. In all sections, the level directed by the WT miR-22 promoter was set to 1. The double asterisk indicates a statistically significant difference ( P <0.001, Student's t -test). Full size image To investigate further the influence of transcription initiation rate directed by the A20 promoter on productive miRNA synthesis, we utilized a previously characterized TATA-box version of this promoter (A20-TATA) [19] . The A20-TATA is more active than the native A20 and the miR-22 promoters ( Fig. 6c , black bars). We next assessed the efficiency of miRNA synthesis under the control of the different promoters by northern blot ( Fig. 6c , grey bars). While the relative level of miRNA expression directed by miR-22 and A20 promoters correlates well to that of the luciferase activity, the A20-TATA promoter, which is 3.5- and 1.5-fold stronger than the A20 and miR-22 promoters, respectively, directs only slightly higher levels than the A20 promoter and 2.5-fold lower miRNA levels compared with miR-22 promoter ( Fig. 6c ). This finding further confirms that miRNA synthesis is not compatible with transcription occurring through re-initiation. Similar findings were observed with the TATA box containing miR-375 promoter ( Supplementary Fig. S4 ). Influence of initiation rate on miR-146 induction by NF-κB The failure to efficiently induce exogenous miRNA by NF-κB may have implications on productive expression of native miRNA targets of NF-κB. To investigate this possibility, we monitored the expression of the NF-κB-dependent miR-146a , which is expressed in a subset of cell types, and is part of a negative feedback mechanism controlling NF-κB in these cells [36] , [37] . THP-1 monocytic cells were challenged with lipopolysaccharide (LPS) and harvested at various time points after induction to detect the emergence of the primary transcript. We designed gene-specific primers for reverse transcription and qPCR amplification from the first exon, which reflects NF-κB induction level and promoter strength, and three sets from the second exon: one from the 5′-end of the exon, the second immediately downstream, from the stem and loop region and the third corresponds to the processed pre-miRNA [38] , as shown schematically in Fig. 7a . The second exon is located ~16 kb from the beginning of the gene. If elongation is not interrupted the induction fold at the first and the second exon should be similar but in case of premature termination a decrease in induction rate is expected. As shown in Fig. 7b , induction of the primary transcript derived from the first exon ( a product) is initially detected 60 min after LPS addition, and is further increased after 2 h. The induction of the primary transcript from the beginning of the second exon ( b product) is highly similar to the a product, indicating normal progress of transcription between these positions. Interestingly, the induction of the c and d segments located few nucleotides downstream from the b product and encoding the miR-146a, is delayed and starts to appear only 120 min after LPS treatment. Moreover, their induction fold is lower compared with that seen from the same exon just upstream, reminiscent of an elongation defect ( Fig. 7b ). The observed elongation interference near the miRNA site may be even more pronounced if we take into account that pri-miRNA, represented by the a , b and c segments, is the first to be cleaved during miRNA biogenesis and has a shorter half-life compared with the mature miRNA [29] , [30] , [31] . The delay in the induction is also reflected in the levels of the mature miR-146a ( Fig. 7b , upper graph) in spite of its remarkable long half-life of ~200 h (ref. 39 ). 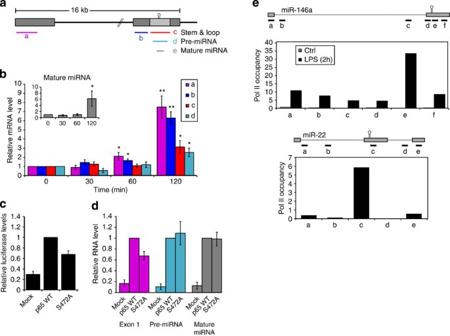Figure 7: Reduced efficiency of miR-146a and miR-22 synthesis is associated with PolII pausing. (a) A schematic representation of themiR-146agene and the location of the primers used for transcript analysis. (b) THP-1 cells were induced with LPS for the indicated times. Gene-specific reverse transcription (RT) was carried out with primers whose positions are schematically shown on theapanel. The RT reaction also included primers forGAPDHas normalizing control. Another set of primers was used to amplify the mature miR-146a as described in the Methods. PCR amplification included controls without reverse transcriptase to ensure lack of contaminating genomic DNA. The results represent the mean of 3–6 independent experiments. Error bars represent s.e. The value of the transcripts of each amplicon before LPS induction (time 0) was set to 1. * and ** indicate significant change (P<0.05 or 0.005, respectively using Student’st-test) relative to time=0. (c) HEK293T cells were transfected with theA20 luciferasereporter gene together with either the wild-type p65 or the S472A mutant. The results represent the mean of three independent experiments. Error bars represent s.e. The activity of the wild-type p65 was set to 1. (d) THP-1 cells were transfected with the wild type or the S472A mutant of p65. At 48 h after transfection levels ofmiR-146awere measured using RT–qPCR with primers from the first exon (initiation rate) and the pre and mature miR as shown schematically ina. The results represent the mean of 3 independent experiments. Error bars represent s.e. The activity of the wild-type p65 was set to 1. (e) The regions encodingmiR-146aandmiR-22are strong PolII pause sites. Upper panel: THP-1 cells were induced by LPS for 2 h and subjected to chromatin inmmunoprecipitation (ChIP) assay using PolII antibodies followed by qPCR. The amplicons, representing different regions of the genes, were normalized to the input and control antibodies. Lower panel: HeLa cells were subjected to ChIP assay with PolII antibodies followed by qPCR analysis using primers from various positions of themiR-22gene. The results are normalized to the input and control antibodies. Figure 7: Reduced efficiency of miR-146a and miR-22 synthesis is associated with PolII pausing. ( a ) A schematic representation of the miR-146a gene and the location of the primers used for transcript analysis. ( b ) THP-1 cells were induced with LPS for the indicated times. Gene-specific reverse transcription (RT) was carried out with primers whose positions are schematically shown on the a panel. The RT reaction also included primers for GAPDH as normalizing control. Another set of primers was used to amplify the mature miR-146a as described in the Methods. PCR amplification included controls without reverse transcriptase to ensure lack of contaminating genomic DNA. The results represent the mean of 3–6 independent experiments. Error bars represent s.e. The value of the transcripts of each amplicon before LPS induction (time 0) was set to 1. * and ** indicate significant change ( P <0.05 or 0.005, respectively using Student’s t -test) relative to time=0. ( c ) HEK293T cells were transfected with the A20 luciferase reporter gene together with either the wild-type p65 or the S472A mutant. The results represent the mean of three independent experiments. Error bars represent s.e. The activity of the wild-type p65 was set to 1. ( d ) THP-1 cells were transfected with the wild type or the S472A mutant of p65. At 48 h after transfection levels of miR-146a were measured using RT–qPCR with primers from the first exon (initiation rate) and the pre and mature miR as shown schematically in a . The results represent the mean of 3 independent experiments. Error bars represent s.e. The activity of the wild-type p65 was set to 1. ( e ) The regions encoding miR-146a and miR-22 are strong PolII pause sites. Upper panel: THP-1 cells were induced by LPS for 2 h and subjected to chromatin inmmunoprecipitation (ChIP) assay using PolII antibodies followed by qPCR. The amplicons, representing different regions of the genes, were normalized to the input and control antibodies. Lower panel: HeLa cells were subjected to ChIP assay with PolII antibodies followed by qPCR analysis using primers from various positions of the miR-22 gene. The results are normalized to the input and control antibodies. Full size image The lower level of stimulation seen for the pre-miRNA segments 60 and 120 min after induction can be explained by premature termination, which may lead to loss of some initiation events. According to this possibility, reducing the rate of initiation by NF-κB is expected to increase the efficiency of miRNA synthesis as observed for the miR-22 ( Fig. 6a ). To test this idea, we utilized a mutant of the NF-κB protein p65, S472A, which was identified in a screen of mutants within the p65 activation region. This mutant displays reduced activation potential compared with the wild-type protein in reporter gene assay ( Fig. 7c ). THP-1 cells were transfected with the wild type and the S472A mutant of p65 and the influence of these variants on the levels of the endogenous miR-146a was monitored. The transcript level measured from the first exon, which reflects the initiation rate, is induced by both p65 variants but the activation by the S472A mutant is reduced to same extent as in the reporter assay ( Fig. 7d , pink columns). Remarkably, the induced levels of the pre-miR-146a as well as the mature miR-146a are comparable ( Fig. 7d , blue and grey columns). These results suggest that the efficiency of miRNA synthesis conferred by the S472A mutant is higher than the wild-type p65. Together, the results with the exogenous and endogenous miRNA induction by NF-κB support the idea that transcription elongation through an obstruction in the form of a miRNA is less productive when the rate of transcription initiation is high. As miR-146a is part of a negative feedback mechanism controlling NF-κB activation [36] , [37] , the postponement of its induction along with its slower accumulation is likely to allow a time frame for NF-κB to function before its activity is terminated by high levels of miR-146a. Transcriptional pausing at miRNA sites A possible explanation for the incompatibility of high initiation frequency with productive miRNA synthesis is strong pausing of PolII at the miRNA site. High initiation frequency is likely to result in crowding of PolII near the pause site, which may lead to collision. To test whether the region encoding the miRNA is a pause site, we used chromatin inmmunoprecipitation assay to examine PolII occupancy along the miR-146a gene, in untreated and LPS-induced THP-1 cells and along miR-22 gene in HeLa cells ( Fig. 7e ). As PolII stays longer at pause sites, we expect its levels to be higher at these sites. In both miR-146a and miR-22 genes, the level of PolII near the promoter is relatively high and is gradually decreased in the body of the gene, including the positions located very close to the pre-miRNA site. The levels of PolII at the miRNA site however, are remarkably high compared with all other upstream and downstream regions ( Fig. 7e ). These findings confirm the prediction that the regions encoding the miRNA compose a strong pause site for PolII. RNA synthesis is a multi-step process that starts with transcription initiation, proceeds with transcription elongation, and ends with processing of the primary transcript. While the connections between transcription elongation and mRNA processing are well established, much less is known about the links between transcription initiation and elongation. We demonstrate here that an important determinant that influences the efficiency of miRNA expression is the mechanism of transcription initiation. By modulating the transcription initiation rate up and down for exogenous and endogenous miRNAs, we found that miRNA synthesis is less efficient when the initiation rate is increased through a TATA box or NF-κB, but becomes more productive when the frequency of initiation is reduced. Combining the observations that TATA box and NF-κB allow efficient re-initiation ( Fig. 5 , Supplementary Fig. S3 and Yean and Gralla [32] and Ainbinder et al . [35] ) and that the miRNA is a strong pause site for PolII ( Fig. 7 ), we propose that transcription re-initiation causes crowding of PolII at the miRNA site, leading to collision of PolII molecules and premature termination ( Fig. 8 ). While the data accumulated in this study are consistent with this model, other mechanisms may also contribute to this phenomenon. 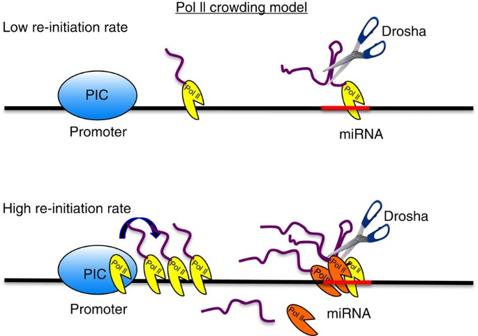Figure 8: PolII crowding model. TATA and NF-κB promote transcription re-initiation, resulting in local crowding of PolII running together. Co-transcriptional miRNA processing pauses PolII, leading to a ‘traffic-jam’, which causes some of the following PolII molecules to abort. Consequently, the efficiency of miRNA synthesis is reduced. According to this model, slowing the transcription rate will create more ‘traffic jams’ and further decrease of miRNA synthesis. On the other hand, reducing initiation rate increases productive miRNA synthesis. Figure 8: PolII crowding model. TATA and NF-κB promote transcription re-initiation, resulting in local crowding of PolII running together. Co-transcriptional miRNA processing pauses PolII, leading to a ‘traffic-jam’, which causes some of the following PolII molecules to abort. Consequently, the efficiency of miRNA synthesis is reduced. According to this model, slowing the transcription rate will create more ‘traffic jams’ and further decrease of miRNA synthesis. On the other hand, reducing initiation rate increases productive miRNA synthesis. Full size image We provide two lines of evidence that a high initiation rate is associated with premature termination in miRNA gene. Reduced miRNA production directed by TATA box is not accompanied with read-through and enhancement of expression of the downstream luciferase ( Fig. 3f ), which was expected if premature termination had not occurred. The second is a decrease in primary miR-146a transcript induction at exactly the pri- and the pre-miRNA boundary ( Fig. 7b ). Transcription elongation rate appears to have differential effect on productive miRNA synthesis as well as on a subset of protein-coding genes in a manner closely correlated with the mechanism of transcription initiation. Through the introduction of a slow elongating form of RNA PolII, we observed a dramatic reduction in productive expression of endogenous and exogenous miRNAs controlled by TATA promoters, supporting the idea that a high rate of transcription initiation, possibly in bursts leads to the observed inefficient production of miRNA. Previous studies reported that high elongation rate is less compatible with alternative splicing, as a slow elongating PolII increased the utilization of weak splicing signals and alternative splicing [23] . In the event that rapid elongation rates are responsible for the inefficient miRNA production, we would have expected the efficiency of the miRNA synthesis to increase with the slow PolII, while it was actually decreased. Our findings are also inconsistent with reduced recruitment of miRNA-processing factors, as we would have expected a different outcome if cleavage of the primary transcript had not occurred ( Fig. 3f ). In addition, the slow PolII, by staying for a longer time at pause sites such as the miRNA region, was expected to increase the efficiency of recruitment of miRNA-processing factors. However, the outcome of the slow polymerase was an even greater decrease in miRNA synthesis. It is therefore anticipated that under certain physiological conditions in which PolII processivity is altered [40] , [41] or transcription re-initiation rate is regulated, [42] the effect on miRNA expression would be differential. Pausing during elongation is not expected to significantly affect miRNA production if the spacing between re-initiation events is longer than the time that PolII stays at pause sites. However, when the waiting time of PolII at pause site(s) is longer than the interval between initiation events, collision between PolII molecules will destroy a fraction of the initiation events ( Fig. 8 ). The average time lapse between re-initiation events in vitro for various TATA promoters and for NF-κB-driven transcription was calculated to be ~2–10 min [32] , [35] , [42] . RNA counting in single living bacterial and eukaryotic cells revealed that individual initiation events in vivo are similarly spaced apart in a range of few minutes [43] , [44] , [45] . We therefore infer that the duration of pausing at the miRNA sites, has to be longer than the rate of re-initiation directed by a TATA box, and can be estimated to last several minutes. This is a surprisingly prolonged pausing for PolII, but in most cases this delay is not expected to affect the steady-state levels of miRNAs, as the promoters driving them usually direct dispersed initiation events. The lengthy pausing calculated here is consistent with the reported slow kinetics of co-transcriptional miRNA processing by the microprocessor [5] . Pausing at the pre-miRNA may be important for its appropriate folding, reminiscent of the pausing at riboswitches of bacteria, which was proposed to provide a time window for the RNA to fold without interference of competing sequences present downstream [46] , [47] . The findings reported here are likely to have implications that extend beyond miRNA genes, in particular for those genes containing a TATA-box promoter along with transcriptional pause site(s). A prime candidate for this class is the gene set identified here that have short length but was nevertheless downregulated when transcription elongation rate was reduced. It is possible, that the effect of the slow polymerase on their expression is similar to that observed with the miRNAs. The results of this study may also be the basis to explain why TATA-box genes tend to be short and more sensitive in their expression to gene length [14] . This also may be related to the high frequency of transcription initiation and the increased probability that PolII will encounter an obstacle during elongation with increased gene length. In contrast, when initiation is less frequent the distance between each PolII molecule allows sufficient time for PolII to deal with the block, and to avoid collision with the succeeding PolII molecules. In summary, the transcriptional features of miRNA genes presented here suggest that miRNAs are remarkable strong pause sites that challenge the robustness of PolII, which generally can transcribe very long genes without dissociation. When the flow of polymerases on a miRNA gene is very high, collision between PolII molecules is inevitable, resulting in premature termination ( Fig. 8 ). Plasmid construction The promoters of miR-22, A20 WT, A20 TATA, miR-375 WT and miR-375 TATA mutant were previously described [19] , [24] , [48] . For generation of miR-22-TATA promoter mutant, a PCR fragment bearing the TATA-box mutation was cloned between Pvu II and Hin dIII sites of the promoter. The primers used are shown in Supplementary Table S2 . To construct the MG, we first amplified a genomic fragment containing 487 bp upstream and 150 bp downstream to the miR-22 TSS and inserted it into pGL2 basic (Promega) between Sma I and Hin dIII sites. This fragment contains the miR-22 promoter, the first exon and the 5′-end of the first intron. This construct was then used as a backbone for insertion of a second fragment from the 3′-end of the miR-22 first intron up to the end of the second exon. The second fragment was inserted between Xho I and Hin dIII sites. The MG was then amplified and cloned in front of the miR-22-TATA, A20 WT and A20 TATA promoters using cleavage and fill-in to create a blunt end downstream to the promoter, and an Eco RI site from the luciferase gene. The MG constructs were cleaved with Hin dIII and self-ligated to create the MG Δpre constructs. The primers used for these constructions are shown in Supplementary Table S2 . To generate the MG under the miR-375 WT and TATA-mutant promoters, the miR-375 promoter variants were amplified by PCR and then replaced the miR-22 promoter through Sma I and Eag I restriction sites. Primers used to amplify the miR-375 WT and miR-375 TATA-mutant promoters are shown in Supplementary Table S2 . Internal control for the small RNA northern blots was created by insertion of double-stranded oligonucleotide ( Supplementary Table S2 ) into the pSUPER plasmid between the Bgl II and Sal I sites. The α-amanitin-resistant PolII constructs were previously described [23] and generously provided by A.R. Kornblihtt (University of Buenos Aires, Argentina). To create the DTIE deletion, we used the full MG as a template. PCR was used to amplify the fragment just downstream to the DTIE up to the lucifearse gene (see Supplementary Table S2 for primers). This fragment was then inserted between the Eag I and Eco RI sites. The S472A mutant of p65 was generated through the RF-cloning technique [49] using the primers shown in Supplementary Table S2 . Cells and transfections HEK293T and hamster pancreatic HIT cell lines were maintained in DMEM supplemented with 10% fetal calf serum. THP-1 cells were maintained in RPMI-1640 and 10% fetal calf serum. Transfection into HEK293T cells was done using the CaPO 4 method [19] . For reporter gene assay, cells were harvested 24 h after transfection. For northern blot assays, RNA was extracted 48 h after transfection. For the slow polymerase experiments, cell medium was changed 24 h after transfection with fresh medium containing 10 μg ml −1 α-amanitin (Apollo Scientific). HIT and THP-1 cells were transfected using Jet-PEI reagent (Polyplus Transfection). Chromatin immunoprecipitation THP-1 cells that were induced by LPS for 2 h and HeLa cells (~1.5 × 10 6 for each IP) were crosslinked with 1% formaldehyde for 10 min at room temperature. Then chromatin extract was prepared followed by immunoprecipitations with either general Pol II antibody (S-20 from Santa Cruz Biotechnology) or control serum. DNA samples were analysed by qPCR in an ABI 7300 Real-Time PCR system using Power SYBR PCR reaction mix (ABI). Primer sequences are shown in Supplementary Table S2 . RNA analyses For gene expression profiling, we used the GeneChip human Gene 1.0 ST Array (Affymetrix). Hybridizations were performed at the Microarray unit at the Weizmann Institute of Science. One microgram of total RNA from each sample (Rpb1-am r and R749H-am r ), from three independent experiments, was labelled. Microarray data analysis was performed by the Bioinformatics unit at the Weizmann Institute of Science. Data were first normalized using GC-RNA. Results are expressed as a log2 of the ratio between Rpb1-am r and R749H-am r . Genes with intensity greater than 4.5 and a fold change greater than 1.2 in all three replicates were considered significant. For northern blot assay of small RNA, total RNA was extracted from HEK293T or HIT cells with Tri-reagent (MRC Inc.). Total RNA (5–10 μg) was loaded onto a 15% acrylamide gel and run at 180 V for 90 min, in 1 × TBE. RNA was then transferred from the gel to a GeneScreen-Plus membrane (NEN), at 200 mA for 2 h, in 0.5 × TBE. Next, the RNA was crosslinked to the membrane with UV irradiation. Pre-hybridization was carried out at 42 °C for 2 h in hybridization buffer (5 × SSC, 20 mM Na 2 HPO 4 (pH 7.2), 7% SDS and 2 × Denhardt’s solution), after which the 32 P-labelled probe ( Supplementary Table S2 ) was added. Hybridization was carried out 16–24 h at 42 °C. The membrane was then washed three times at 42 °C with 3 × SSC, 25 mM NaH 2 PO 4 (pH 7.5), 5% SDS and 10 × Denhardt’s solution. Hybridization products were visualized using phosphoimager (Fuji, BAS 2500). For northern blot analysis of mRNA, total RNA (15 μg) was loaded onto a 1% agarose gel containing 1 × MOPS and 1% formaldehyde, and run at 90 V for 3 h, in 1 × MOPS. The gel was subjected to capillary transfer to a GeneScreen-Plus membrane (NEN). RNA was crosslinked to the membrane by UV irradiation. Pre-hybridization was carried out at 42 °C for 2–4 h in hybridization buffer (2 × SSC, 50% formamide, 1% SDS, and 5 × Denhardt’s solution and 100 μg ml −1 salmon sperm DNA), after which the 32 P-labelled GFP or luciferase probes were added for 16–24 h hybridization at 42 °C. The membrane was then washed five times with 2 × SSC and 0.1% SDS solution and once with 0.2 × SSC and 0.1% SDS, at 42 °C. For quantitative RT–PCR of miR-146a primary transcript,THP-1 cells were treated with LPS (100 ng ml −1 ) for 0, 10, 30, 60 or 120 min followed by total RNA preparation. Gene-specific cDNA was then prepared from 5 μg of total RNA, using SuperScript II reverse transcriptase (Invitrogene). The real-time PCR was performed with 20 μl tubes in the ABI 7300 Real-Time PCR system and analysed by the manufacturer provided System Software and normalized with GAPDH. Analysis of genes affected by the slow PolII shown in Fig. 1 was done in a similar way. Primer sequences are shown in Supplementary Table S2 . For quantitative analysis of endogenous miRNAs, the RNA extracted from α-amanitin-selected cells was used to create complementary DNA using the miScript reverse transcription kit (Qiagen). miRNA levels were measured by qPCR with the U6 gene as an internal control. The primer sequences are shown in Supplementary Table S2 . In vitro transcription assays and 5′RACE Nuclear extract used for in vitro transcription assays was prepared using the salt extraction method [35] . Assembly of in vitro transcription reaction was conducted in a total volume of 18 μl containing 9 μl of nuclear extract in a buffer consisting of 100 mM KCl, 20 mM HEPES (pH 7.9), 2 mM MgCl 2 , 20% glycerol and 1 mM dithiothreitol, 200 ng of plasmid carrying either WT or TATA-box containing miR-22 promoter and 100 ng of GFP plasmid directed by the CMV promoter. The mixture was incubated at 30 °C for 30 min to allow PIC formation. Transcription was initiated by the addition of 2 μl of nucleotide solution containing 5 mM ATP, GTP, CTP and UTP. The reaction was terminated after 10 min by the addition of 100 μl of stop solution (0.2 M NaCl, 20 mM EDTA, 1% sodium dodecyl sulphate, 0.25 mg ml −1 yeast tRNA, 50 μg ml −1 proteinase K) and incubation at room temperature for 2 min. To inhibit re-initiation, Sarkosyl was added to the reaction mixture 2.5 min after initiation. The RNA was extracted with phenol-chloroform (1:1) and then with chloroform and then precipitated with ethanol. The RNA products were then used as a template to create cDNA with superscript II (Invitrogen) according to the manufacturer’s instructions, using Luciferase and GFP-specific primers (see Supplementary Table S2 ). The cDNA was purified using PCR purification kit (Qiagen), followed by addition of polyG to the 5′-end using TdT enzyme (Promega) for 1 h at 37 °C. The reaction was terminated by heat inactivation for 15 min at 65 °C, and the products were purified with the PCR purification kit (Qiagen). The modified cDNA was used as a template for PCR using nested reverse primers from the luciferase and GFP genes, and primers spanning the exact TSS of each template as forward primers ( Supplementary Table S2 ). PCR products were run on 6% polyacrylamide gel. Accession Codes: The microarray data have been deposited in Gene Expression Omnibus under series accession code GSE48163 . How to cite this article: Marbach-Bar, N. et al . Disparity between microRNA levels and promoter strength is associated with initiation rate and Pol II pausing. Nat. Commun. 4:2118 doi: 10.1038/ncomms3118 (2013).